Nanoporous frameworks exhibiting multiple stimuli responsiveness Nanoporous frameworks are polymeric materials built from rigid molecules, which give rise to their nanoporous structures with applications in gas sorption and storage, catalysis and others. Conceptually new applications could emerge, should these beneficial properties be manipulated by external stimuli in a reversible manner. One approach to render nanoporous frameworks responsive to external signals would be to immobilize molecular switches within their nanopores. Although the majority of molecular switches require conformational freedom to isomerize, and switching in the solid state is prohibited, the nanopores may provide enough room for the switches to efficiently isomerize. Here we describe two families of nanoporous materials incorporating the spiropyran molecular switch. These materials exhibit a variety of interesting properties, including reversible photochromism and acidochromism under solvent-free conditions, light-controlled capture and release of metal ions, as well reversible chromism induced by solvation/desolvation. Stimuli-responsive molecules [1] or nanoparticles [2] are capable of changing their structure and/or properties in response to external stimuli such as small molecules, light or magnetic field. These entities have recently attracted much attention as key components of stimuli-responsive materials, examples of which include self-darkening windows [3] , self-healing coatings [4] , [5] , [6] , or silica-based delivery vesicles, which can be engineered to release cargo molecules upon activation with a variety of external stimuli [7] , [8] . Among these different stimuli, light is arguably the most attractive: it is a stimulus that can be delivered instantly, into a precise location, and in the form of different wavelengths, to which different photoresponsive molecules selectively respond [9] , [10] , [11] . One of the most unique examples of molecular switches is spiropyran, whose closed-ring, hydrophobic SP isomer transforms into a highly polar, open-ring merocyanine (MC) form upon exposure to ultraviolet light, whereas the reverse reaction can be induced by visible light [12] , [13] , [14] . Moreover, this reversible isomerization can be triggered by a variety of other external stimuli, such as acids and bases, metal ions, temperature, redox potential and mechanical force. The isomerization process, however, entails a large change in the conformation of the molecule—an obstacle as far as efficient isomerization within solid-state materials is concerned. In order to efficiently switch, spiropyran molecules require conformational freedom, which usually is not available within the densely packed arrays of molecules in the crystalline state. An attractive way to satisfy this conformational freedom requirement would be to harbour the spiropyran moieties within the nanopores of porous aromatic frameworks (PAFs)—a recently introduced [15] , [16] , [17] family of microporous polyphenylene materials. This strategy could not only enable efficient isomerization of spiropyran in the solid state, but it would also allow for the control of the beneficial properties of PAFs (such as storage of gaseous cargo) using external stimuli. Here we describe two strategies ( Fig. 1 ) to construct stimuli-responsive nanoporous materials based on spiropyran: the first approach is based on a three-component Suzuki coupling reaction involving (i) a rigid, tetratopic boronic acid 4 , (ii) a rigid, tetratopic bromide 3 , and (iii) a photoresponsive, monotopic bromide 1 . We refer to the products of this route as PhotoPAF- χ SP (photoresponsive porous aromatic framework), where χ SP indicates the extent of spiropyran loading. Second, we consider a two-component coupling between the boronic acid 4 and a rigid photoresponsive ditopic bromide 2 —here, the resulting material is found to have a significantly more flexible structure, hence, we refer to it as photoresponsive porous aromatic network or PhotoPAN. Both types of materials—PhotoPAFs and PhotoPAN—exhibit a variety of interesting properties, including light-controlled capture and release of metal ions, examples of reversible photochromism and acidochromism of spiropyran under solvent-free conditions, as well as reversible chromism induced by solvation/desolvation. 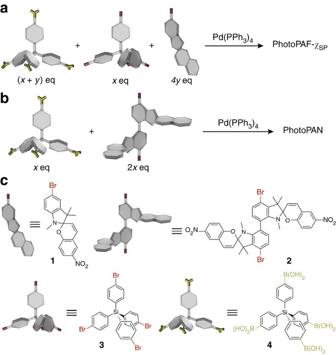Figure 1: Two strategies to prepare nanoporous materials incorporating spiropyran. (a) Preparation of photoresponsive porous aromatic framework (PhotoPAF). (b) Preparation of photoresponsive porous aromatic network (PhotoPAN). (c) Structural formulae of the building blocks. Figure 1: Two strategies to prepare nanoporous materials incorporating spiropyran. ( a ) Preparation of photoresponsive porous aromatic framework (PhotoPAF). ( b ) Preparation of photoresponsive porous aromatic network (PhotoPAN). ( c ) Structural formulae of the building blocks. Full size image Synthesis of nanoporous materials incorporating spiropyran Both PhotoPAFs and PhotoPAN were synthesized via Pd-catalysed Suzuki cross-coupling reactions (see Supplementary Figs 1–28 and Supplementary Methods for the synthesis and characterization of all small molecules). In a typical procedure, a single-neck round-bottom flask was charged with a mixture of bromide and boronic acid precursors, K 2 CO 3 and a catalytic amount of Pd(PPh 3 ) 4 were added, and the reactants were heated under a blanket of nitrogen in a 1:1 tetrahydrofuran (THF)–water solvent mixture at 75 °C for 2 days. In the case of PhotoPAFs, precursors 1 , 3 and 4 were used in ratios such that the total number of bromide groups (in 1 and 3 ) was equal to the number of boronic acid functionalities (in 4 ; see Fig. 1; we used Si-based, as opposed to C-based, building blocks 3 and 4 as they are easily prepared from commercially available starting materials [18] , [19] ). For PhotoPAN, a 2:1 mixture of precursors 2 and 4 was used ( Fig. 1 ). The solids that precipitated during the reaction were collected, washed extensively with water, acids, bases and various organic solvents, and finally dried in a vacuum oven (see Methods for detailed procedures). We employed a variety of characterization techniques to verify successful incorporation of spiropyran into, and to quantify its loading ( χ SP ) within the nanoporous materials (we define χ SP as the molar ratio of spiropyran in PhotoPAFs to the total ratio of aryl groups originating from starting materials 1 and 3 ). χ SP values were determined by correlating weight percentages of carbon, hydrogen and nitrogen to the composition of the feed mixture as described in Methods. As expected, we found that χ SP was proportional to the percentage of 1 in the initial mixture; however, it was on average only half of the spiropyran content expected from the composition of the feed. This result can be understood based on the fact that 3 has four reactive groups; once one of them reacts, the molecule becomes incorporated in the growing network and the remaining three groups are more likely to react with the –B(OH) 2 groups, which are also part of the existing polymer. Successful coupling reaction as well as the presence of spiropyran in the final material was confirmed by infrared spectroscopy. We followed the progress of the reaction by monitoring the intensity of boronic acid 4 ’s O–H stretching vibrations (the intense band centered at ∼ 3,400 cm −1 ). A nearly complete disappearance of absorption in this region in PhotoPAN and a variety of PhotoPAFs ( Supplementary Fig. 29 ) confirms the high yield of the C–C coupling reaction (residual absorption can be attributed to unreacted boronic acid or to the presence of small amounts of water in the nanopores). The presence and loading of spiropyran, on the other hand, are best appreciated by the peak at ∼ 1,340 cm −1 , which is due to the symmetric stretching mode of the NO 2 group (see Supplementary Fig. 29b ) [20] . To further demonstrate the successful incorporation of spiropyran, we performed 1 H and 13 C solid-state nuclear magnetic resonance (NMR) studies. 1 H magic angle spinning (MAS) NMR spectrum of PhotoPAF-3.6%, for example, shows a major peak centered at δ =8.2 p.p.m., in addition to a smaller one at ∼ 2 p.p.m. ( Supplementary Fig. 30a ). The former can be attributed to protons bound to unsaturated carbon atoms, whereas the latter is due to the spiropyran’s CH 3 protons (and the residual solvent often observed [15] , [21] , [22] in solid-state NMR experiments; we also observed a small peak in this region for a PAF lacking any spiropyran—cf Supplementary Fig. 30d ). As expected, the upfield peak significantly increased in PhotoPAN, as shown in Supplementary Fig. 30b ; interestingly, integrating the ∼ 8 and ∼ 2 p.p.m. signals gives the ratio of ∼ 1.1:1, very similar to the 11:9 stoichiometric ratio of the protons attached to unsaturated versus saturated carbons. Similar trends were found in 13 C spectra, whereby PhotoPAF-3.6% and PhotoPAN showed increasing peaks in the 20–30 p.p.m. region (diagnostic of the spiropyran’s methyl groups, see right panel of Supplementary Fig. 30 ). Finally, the varying amounts of spiropyran were verified by simultaneous thermal gravimetric analysis (TGA)–differential scanning calorimetry (DSC) measurements ( Supplementary Fig. 31 ). Both mass loss (TGA) and differential heat flux (DSC) showed two-step profiles, with a major change at ∼ 550 °C—a signature of the decomposition of the polyphenylene network [15] —accompanied by a minor one at ∼ 350 °C. This latter transition can be attributed [23] to the loss of spiropyran—indeed this transition is absent from spiropyran-free PAF, and it becomes increasingly pronounced as the amount of the switch increases (see Supplementary Fig. 31 ). Finally, we performed several control experiments to verify whether the spiropyran moieties are indeed incorporated covalently within the host PAFs, as opposed to 1 being trapped in the nanopores during the synthesis of the frameworks. First, to demonstrate the activity of the aryl bromide 1 in the Suzuki cross-coupling reaction, we attempted a model coupling between 1 and phenylboronic acid under conditions identical to those employed in the preparation of PhotoPAFs. Successful synthesis and characterization of the coupling product is described in Supplementary Methods (see also Supplementary Figs 26–28 ). Second, as-prepared PhotoPAFs were washed multiple times (see detailed procedure in Methods) to ensure the removal of all residual small molecules. Finally, we performed a two-component coupling involving stoichiometric amounts of 3 and 4 in the presence of the parent spiropyran (1′,3′-dihydro-1′,3′,3′-trimethyl-6-nitrospiro[2 H -1-benzopyran-2,2′-(2 H )-indole])—that is, 1 lacking the bromide group. Following the standard washing procedure, we found no signature of the spiropyran group in any of the characterization techniques described above. 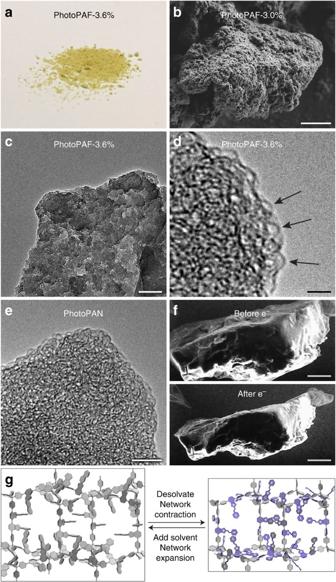Figure 2: Structures of nanoporous materials incorporating spiropyran. (a) Photograph of a macroscopic sample of photoresponsive porous aromatic framework (PhotoPAF)-3.6% (∼100 mg). (b) Scanning electron microscopy image of PhotoPAF-3.0%. (c) Transmission electron microscopy (TEM) image of PhotoPAF-3.6% at a low magnification. (d) TEM image of PhotoPAF-3.6% at a high magnification. Arrows indicate entities that are likely individual nanopores. (e) TEM image of photoresponsive porous aromatic network (PhotoPAN). (f) Structural collapse of PhotoPAN upon prolonged exposure to the electron beam (see alsoSupplementary Movies 1–3). (g) Schematic representation of PhotoPAN network contraction/expansion accompanied by spiropyran ring opening/closing as a result of desolvation/solvation. Scale bars correspond to 5 μm (b), 100 nm (c), 2 nm (d), 5 nm (e) and 50 μm (f). Spiropyran isomerization triggered by desolvation and structural collapse Figure 2 shows typical optical and electron micrographs of our nanoporous materials (see Supplementary Figs 32 and 33 for additional images). As evident from the electron micrographs, the structures of both PhotoPAFs and PhotoPAN lack long-range order, in agreement with previous reports [15] , [24] , [25] on PAFs obtained by irreversible C–C coupling reactions. Still, the porous nature of these materials can easily be discerned by transmission electron microscopy (TEM): focusing on the edge of the sample revealed the presence of ∼ 1 nm nanopores ( Fig. 2d ). Interestingly, inspection of the samples using electron microscopy methods revealed an unexpected difference in the mechanical properties of these two types of materials: when exposed to the electron beam under reduced ( ∼ 10 −5 mBar) pressure typical for the operation of electron microscopes, the structure of PhotoPAN collapsed (cf scanning electron microscopy (SEM) images in Fig. 2f ; see also Supplementary Movies 1–3 ), whereas PhotoPAFs remained unaffected. This collapse can be attributed to the removal of residual solvent molecules from the nanopores of PhotoPAN; the absence of analogous structural changes in PhotoPAFs is likely due to the more rigid nature of their pores (lacking the 2 ‘spacers’). Figure 2: Structures of nanoporous materials incorporating spiropyran. ( a ) Photograph of a macroscopic sample of photoresponsive porous aromatic framework (PhotoPAF)-3.6% ( ∼ 100 mg). ( b ) Scanning electron microscopy image of PhotoPAF-3.0%. ( c ) Transmission electron microscopy (TEM) image of PhotoPAF-3.6% at a low magnification. ( d ) TEM image of PhotoPAF-3.6% at a high magnification. Arrows indicate entities that are likely individual nanopores. ( e ) TEM image of photoresponsive porous aromatic network (PhotoPAN). ( f ) Structural collapse of PhotoPAN upon prolonged exposure to the electron beam (see also Supplementary Movies 1–3 ). ( g ) Schematic representation of PhotoPAN network contraction/expansion accompanied by spiropyran ring opening/closing as a result of desolvation/solvation. Scale bars correspond to 5 μm ( b ), 100 nm ( c ), 2 nm ( d ), 5 nm ( e ) and 50 μm ( f ). Full size image The low pressure under which electron microscopes operate, however, was not essential to induce the structural collapse of PhotoPAN: we observed a shrinking of the grains even during filtration on a Büchner funnel (overall, drying and exposure to the electron beam decreased the volume of the grains by ∼ 80%, comparable to the free volume of other [15] , [26] , [27] porous frameworks). More remarkably, this shrinking was accompanied by a pronounced change in colour from dark yellow to deep blue. The blue colour is the characteristic of MC: the metastable, open-ring isomer of spiropyran (see Fig. 3a ). As previously established [28] , [29] , [30] , [31] , the normally metastable MC moieties can stabilize one another by interacting via a combination of electrostatic, dipolar and π–π interactions [32] ; this stabilization can trigger spontaneous SP→MC transition when the closed-ring SP moieties are brought in close proximity [33] , [34] . The uniqueness of PhotoPAN lies also in the fact that the transition is reversible: when immersed in various solvents (hexane, toluene, dimethylformamide, methanol, etc. ), the particles swelled ( Fig. 2g ) and regained their original dimensions, whereas their colour faded. Both processes are fast: PhotoPAN resolvated and the colour faded within only a few seconds, whereas shrinking and colouration took less than a second. Moreover, as the transition was not induced by light, the spiropyran switch exhibited excellent reversibility: even after performing 200 solvation–desolvation cycles, we saw no signs of degradation of the switch. 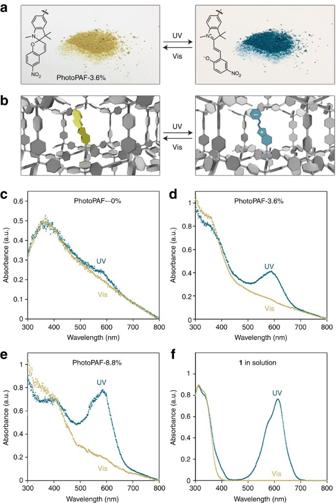Figure 3: Optical properties of PhotoPAFs. (a) Visual changes to PhotoPAF-3.6% upon exposure to low-intensity ultraviolet light. (b) Schematic representation of efficient isomerization of spiropyran inside the nanopores. (c–e) Ultraviolet–visible spectra of suspensions of PhotoPAFs (in 1:1 PhMe-CHCl3) containing different amounts of spiropyran before and after ultraviolet irradiation. PhotoPAF∼0% (c) indicates a sample with a nitrogen content below the detection limit of the available elemental analyser. Integration of the merocyanine peak allows us to determine the composition of the sample as PhotoPAF-0.5%. (f) Ultraviolet–visible spectra of a toluene solution of1before and after ultraviolet irradiation. Vis, visible. Figure 3: Optical properties of PhotoPAFs. ( a ) Visual changes to PhotoPAF-3.6% upon exposure to low-intensity ultraviolet light. ( b ) Schematic representation of efficient isomerization of spiropyran inside the nanopores. ( c – e ) Ultraviolet–visible spectra of suspensions of PhotoPAFs (in 1:1 PhMe-CHCl 3 ) containing different amounts of spiropyran before and after ultraviolet irradiation. PhotoPAF ∼ 0% ( c ) indicates a sample with a nitrogen content below the detection limit of the available elemental analyser. Integration of the merocyanine peak allows us to determine the composition of the sample as PhotoPAF-0.5%. ( f ) Ultraviolet–visible spectra of a toluene solution of 1 before and after ultraviolet irradiation. Vis, visible. Full size image The absence of the MC form within the solvated PhotoPAN was confirmed by ultraviolet–visible spectroscopy: we observed no peak at ∼ 550 nm in optical spectra of the PhotoPAN suspensions in solvents of different polarities (for example, acetonitrile, THF, toluene). At the same time, the formation of MC could be induced by exposing the samples to low-intensity ultraviolet radiation ( λ =365 nm; I =0.7 mW cm −2 ; Supplementary Fig. 34 ), and the resulting blue suspensions faded spontaneously with kinetics characteristic of those of small-molecule spiropyrans in hydrophobic solvents—in other words, ‘normal’ photochromism of spiropyran was observed in all solvents investigated. This finding is in contrast to previous reports on small-molecule spiropyrans, where the equilibrium between the SP and MC isomers was strongly dependent on the polarity of the solvent [32] , [35] (solvatochromism; for example, the relatively polar acetonitrile typically stabilizes the MC form). We find, however, that the aromatic character of the network backbone has a ‘buffering’ effect on the photoswitch, favouring the closed-ring SP isomer irrespective of the solvent. Efficient isomerization of spiropyran in the solid state Although spiropyran within the solvent-free PhotoPAN was permanently ‘frozen’ in the MC state, its solid-state photoisomerization could readily be accomplished when within the nanopores of the more rigid PhotoPAFs. As Fig. 3a shows, for example, when the yellow powder of PhotoPAF-3.6% was exposed to low-intensity ultraviolet light, it turned deep blue within ∼ 3 min, indicative of SP→MC isomerization (see also Supplementary Fig. 35 ). Such efficient photoisomerization at room temperature and under solvent-free conditions is, to our knowledge, unprecedented: although solid-state isomerization of other molecular photoswitches has been reported [36] , [37] , [38] , the significant conformational difference between the closed- and the open-ring isomers of spiropyran has effectively prohibited the long-sought [39] , [40] , [41] photoisomerization of this class of molecules in the solid state. The MC peak was clearly visible at ∼ 590 nm in the optical spectra recorded on suspensions of different PhotoPAFs; in addition, as Fig. 3c–e shows, ultraviolet–visible spectroscopy served as yet another way to demonstrate the control over spiropyran loading: the ∼ 590 nm peak grew with increasing amounts of the photoswitch within the PhotoPAFs. The MC-functionalized PhotoPAFs slowly (within several hours) faded as MC isomerized back to SP in a reaction that could be accelerated (to around a minute) with visible light. These photoirradiation experiments confirmed the rigid nature of PhotoPAFs: we saw (by SEM) no noticeable differences in the size and shape of the samples before and after exposure to ultraviolet and then visible light. Covalent immobilization of spiropyran units prevents them from interacting with one another, which is important in the context of reversible isomerization. As previously established [42] , [43] , irreversible reactions between excited spiropyran molecules are the primary cause of fatigue—that is, gradual degradation of a molecular switch as a result of reversible photoisomerization. This ‘bimolecular’ pathway, however, is greatly inhibited in PhotoPAFs; indeed, we found that deoxygenated (purged with argon) PhotoPAF-3.6% was virtually fatigue-free and no indication of photodegradation could be seen even after performing 100 switching cycles (one cycle=1 min of ultraviolet, I =0.7 mW cm −2 , followed by 1.5 min of visible light, fluorescent bulb I =1.0 mW cm −2 ). In air, however, the ‘monomolecular’ (oxygen-dependent) degradation pathway was still functional [44] , [45] , leading to significant fatigue effects as reported in prior literature [46] . Photoswitchable fluorescence An interesting feature of the spiropyran switch is that while its closed-ring, SP isomer is practically non-fluorescent, MC shows an intense red emission [47] , [48] . Consequently, being able to reversibly photoisomerize under solvent-free conditions, PhotoPAFs showed unique solid-state photoswitchable fluorescence, as shown in Fig. 4a . The intense red emission not only confirms a successful SP→MC isomerization, but also implies that the MC units within the ultraviolet-irradiated PhotoPAFs do not interact with one another; we note that MC–MC stacking leads to fluorescence quenching as reported earlier in the literature [49] , and as manifested by the properties of solid-state PhotoPAN, which, despite featuring spiropyran in the MC form without any ultraviolet irradiation, showed no measurable emission. 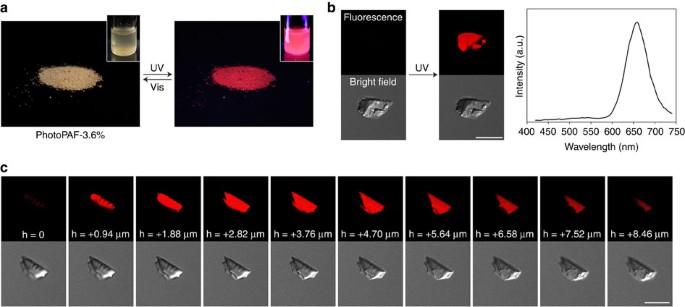Figure 4: Photoswitchable fluorescence in PhotoPAFS. (a) Visual changes to the sample in the solid state and in a toluene suspension (insets) as a result of ultraviolet irradiation. Images on the left were taken under ambient light. Images on the right were taken in the dark under 365 nm illumination. (b) Using ultraviolet to ‘turn on’ fluorescence of a single PhotoPAF-3.6% grain. Also shown is an emission spectrum (excitation wavelength=405 nm) of the same grain. (c) Confocal fluorescence micrographs of a ultraviolet-activated PhotoPAF-3.6% grain focused on different planes along the optical axis of the microscope. Scale bars correspond to 20 μm. Figure 4b shows photoswitchable fluorescence of a single particle of PhotoPAF-3.6% investigated using fluorescence microscopy (see also Supplementary Movie 4 ), along with a typical emission spectrum recorded on the same particle ( λ max =660 nm). We also employed confocal fluorescence microscopy to verify that no phase separation occurs during the synthesis of PhotoPAFs (phase separation could take place if aryl bromides 1 and 3 reacted with the boronic acid 4 with vastly different kinetics). Optical sections acquired over a range of specimen planes (for example, Fig. 4c ) show no preferential accumulation of the fluorescent component at the centre or at the periphery of the grains. Figure 4: Photoswitchable fluorescence in PhotoPAFS. ( a ) Visual changes to the sample in the solid state and in a toluene suspension (insets) as a result of ultraviolet irradiation. Images on the left were taken under ambient light. Images on the right were taken in the dark under 365 nm illumination. ( b ) Using ultraviolet to ‘turn on’ fluorescence of a single PhotoPAF-3.6% grain. Also shown is an emission spectrum (excitation wavelength=405 nm) of the same grain. ( c ) Confocal fluorescence micrographs of a ultraviolet-activated PhotoPAF-3.6% grain focused on different planes along the optical axis of the microscope. Scale bars correspond to 20 μm. Full size image Acidochromism induced by gaseous signals Next, we hypothesized that the switchable moieties located within the nanopores could be actuated by gaseous signals ( Fig. 5a; in solution, MC’s phenoxide anion undergoes protonation upon the addition of strong acids, resulting in a yellow-coloured MCH + species [50] ; see also Supplementary Fig. 34 ). To test our hypothesis, we passed gaseous HCl through a pad of solid PhotoPAN and observed a slow colour change from deep blue to bright yellow ( Fig. 5b ). The seemingly complete disappearance of the initial dark colour suggests a high yield of the MC→MCH + conversion. The protonation reaction was reversible: gaseous NH 3 abstracted protons from MCH + and re-generated the deeply coloured MC-functionalized PhotoPAN. Interestingly, the two processes differed significantly in their kinetics: although protonation occurred gradually over the course of ca 5 min, deprotonation was nearly instantaneous (see Supplementary Movie 5 ). Given that the van der Waals radii of HCl and NH 3 are very similar, such significant discrepancies should be attributed to the differences in reaction kinetics rather than different diffusion coefficients. Overall, these results demonstrate that despite its collapsed structure, MC-rich PhotoPAN still comprises nanopores large enough to allow for transport of small molecules. An interesting consequence of the alternate infusion of HCl and NH 3 is the formation of ammonium chloride in the nanopores of PhotoPAN. Each protonation–deprotonation cycle gives rise to a maximum of one equivalent of NH 4 Cl with respect to the number of MC units. An intriguing question that we will address separately concerns the nature of NH 4 Cl formed within the nanopores, whose sizes likely prohibit the formation of a crystalline phase of the salt. 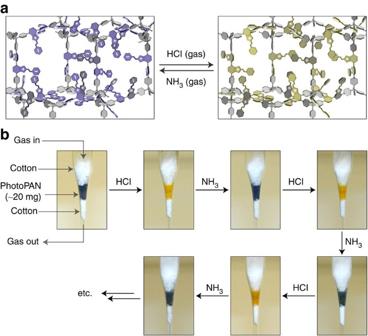Figure 5: Acidochromism of PhotoPAN. (a) Schematic representation of reversible protonation of PhotoPAN induced by gaseous HCl and NH3. (b) Experimental setup used to investigate solid-state acidochromism and demonstration of three cycles of protonation/deprotonation. Figure 5: Acidochromism of PhotoPAN. ( a ) Schematic representation of reversible protonation of PhotoPAN induced by gaseous HCl and NH 3 . ( b ) Experimental setup used to investigate solid-state acidochromism and demonstration of three cycles of protonation/deprotonation. Full size image Light-controlled uptake and release of metal ions Finally, we considered the possibility of employing PhotoPAN as a light-controlled sponge for metal ions. Here, we take advantage of the vastly different affinities of the SP and MC isomers to metal cations: although SP lacks appreciable complexing ability, MC binds metal ions via the phenoxide anions in a 2:1 stoichiometry [51] , [52] . To demonstrate the proof-of-concept, we chose Cu 2+ because of its intense absorption of light in the visible region ( λ max =460 nm for CuCl 2 ·2H 2 O in acetonitrile). Six minutes of sonication with 5 mg of PhotoPAN was sufficient to quantitatively remove Cu 2+ from an acetonitrile solution of 0.4 mg of CuCl 2 ·2H 2 O ( Fig. 6b, d ) in a process that involved Cu 2+ -induced SP→MC isomerization ( Supplementary Fig. 36a ; the ratio we used corresponded to a small excess of SP to Cu 2+ ( ∼ 2.6-to-1; compared with the 2:1 stoichiometric ratio)). As a control experiment, we sonicated the same amount of the copper salt with 5 mg of spiropyran-free PAF (that is, ‘PhotoPAF-0%’), and observed negligible absorption of Cu 2+ even after 30 min of sonication ( Supplementary Fig. 36b ). Next, we exposed the Cu 2+ -soaked PhotoPAN to visible light ( I =1.0 mW cm −2 ) and observed a gradual release of copper ions ( Fig. 6c, d ). PhotoPAFs containing different amounts of spiropyran behaved similarly to PhotoPAN. Although exposure to light induced a side reaction (the well-known [53] , [54] visible light-induced decomposition of CuCl 2 in acetonitrile) and the absorption of the final supernatant was lower than that of the initial solution (see Supplementary Fig. 36c ), quantitative release of copper was confirmed by energy-dispersive X-ray spectroscopy (EDS), which showed the absence of copper in the final PhotoPAN. 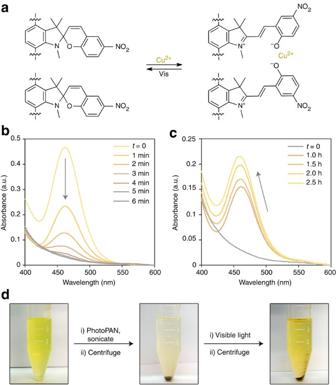Figure 6: Ionochromism of PhotoPAN. (a) Reversible metal ion/light-induced ring opening/closing. (b) Decrease in optical absorption of Cu2+as a result of trapping inside PhotoPAN. (c) Increase in optical absorption of Cu2+as a result of visible light-induced release. All spectra were recorded on supernatant after centrifugation. (d) Visual changes to the copper salt solution as the copper ions are removed from and then released back to the solution. All experiments shown here were performed using 5 mg of PhotoPAN and 0.4 mg CuCl2·2H2O. Figure 6: Ionochromism of PhotoPAN. ( a ) Reversible metal ion/light-induced ring opening/closing. ( b ) Decrease in optical absorption of Cu 2+ as a result of trapping inside PhotoPAN. ( c ) Increase in optical absorption of Cu 2+ as a result of visible light-induced release. All spectra were recorded on supernatant after centrifugation. ( d ) Visual changes to the copper salt solution as the copper ions are removed from and then released back to the solution. All experiments shown here were performed using 5 mg of PhotoPAN and 0.4 mg CuCl 2 ·2H 2 O. Full size image In summary, we developed two synthetic approaches to spiropyran-based nanoporous materials responsive to multiple types of external stimuli. The two approaches are complementary: one leads to structurally rigid PhotoPAFs—materials that feature efficient spiropyran isomerization and MC fluorescence photoswitching in the solid state. The more flexible PhotoPANs, on the other hand, display solid-state acidochromism, light-controlled trapping and release of metal ions from solution, as well as a novel type of chromism induced by solvation and desolvation of the network. These findings have many interesting implications. First, solid-state photoswitching between two isomers (that is, SP and MC) differing vastly in their polarity is expected to affect the amount of gas (for example, H 2 , CH 4 ) trapped in the nanopores, and hence, it can enable the control of gas sorption using light. Second, the reversible capture and release of metal ions can be transduced into catalytic properties of PhotoPANs (for example, initial experiments show that Cu 2+ -functionalized PhotoPAN is a highly active catalyst for the hydrolysis of bromobenzenes). Third, our studies of acidochromism led to the realization that the nanopores of PhotoPANs can act as templates for the preparation of various materials, ammonium chloride being the first material prepared in these ‘nanoflasks’. Finally, we note that our methodology ( Fig. 1 ) is applicable to other functional nanoporous materials, and it allows for the incorporation of more than one type of functionality. In one direction that we are actively pursuing, a four-component Suzuki coupling leads to frameworks featuring both spiropyran and catalytic moieties: we are investigating the applicability of these materials as a novel family of light-controlled catalysts [55] . General Solution 1 H and 13 C NMR spectra were recorded at room temperature on Bruker 300 and 500 MHz spectrometers (Bruker). Chemical shifts ( δ ) are reported in p.p.m. ; multiplicities are indicated by ‘s’ (singlet), ‘d’ (doublet), ‘t’ (triplet), ‘q’ (quartet), ‘quint’ (pentet), ‘m’ (multiplet) or ‘br’ (broad). Coupling constants ( J ) are reported in Hz. Spectra were referenced to residual chloroform ( 1 H: δ =7.26 p.p.m. ; 13 C: δ =77.00 p.p.m. ), dimethyl sulfoxide ( 1 H: δ =2.50 p.p.m. ; 13 C: δ =39.52 p.p.m.) or dichloromethane ( 1 H: δ =5.32 p.p.m. ; 13 C: δ =53.84 p.p.m.). High-resolution mass spectra were recorded at 60–70 eV on a Waters Micromass Q-TOF spectrometer (ESI, Ar; Waters). Single crystal X-ray data for 1 were collected on a Bruker Appex2 KappaCCD diffractometer (Bruker; Mo Kα, λ =0.71073 Å, graphite monochromator, −10≤ h ≤10, −24≤ k ≤24, −22≤ l ≤22, frame scan width=0.5°, scan speed 1.0° per 20 s, typical peak mosaicity 0.74°, 42,225 reflections collected, 3,870 independent reflections; R -int=0.039). The data were processed with Denzo-Scalepack. Structure of 1 was solved with SHELXS. Full matrix least-squares refinement based on F 2 with SHELXL-97 on 295 parameters with no restraints gave final R 1 =0.0223 (based on F 2 ) for data with I >2 σ ( I ) and R 1 =0.0269 on 8,216 reflections, goodness-of-fit on F 2 =1.030, largest electron density peak=0.406 Å −3 , largest hole=−0.263 Å −3 , see also Supplementary Data 1 . Elemental analyses were performed on a Thermo Scientific FlashEA 1112 organic elemental analyser (Thermo Scientific). Fourier transform-infrared spectroscopy was carried out on a Nicolet 380 infrared spectrometer at 4 cm −1 resolution. The spectra were recorded on finely ground samples ( ∼ 0.2 mg) premixed with ∼ 20 mg of KBr (Fourier transform-infrared grade) and pressed into 7-mm pellets using a manual hydraulic press (Specac). TGA and DSC were performed on an SDT Q600 V8.3 Build 101 simultaneous DSC–TGA instrument operating in dry air in the temperature range 25–800 °C, at a heating rate of 20 °C min −1 . SEM was performed on an ULTRA 55 field emission SEM (Carl Zeiss Microscopy, LLC; Carl Zeiss) as well as on a SUPRA 55VP field emission SEM (Carl Zeiss Microscopy, LLC), both operating at 5 kV. TEM was performed on a CM120 Super Twin TEM (Philips) operating at 120 kV. EDS measurements were carried out on a SUPRA 55VP field emission SEM equipped with an Oxford Instruments EDS detector. Ultraviolet–visible spectra were recorded on a Shimadzu UV-3600 spectrometer (Shimadzu). All ultraviolet–visible spectra of PhotoPAFs/PhotoPAN are averages of at least three individual spectra. For ultraviolet irradiation, we used a 4-W hand-held UV lamp (UVP, LLC; model number UVGL-25; light intensity ∼ 0.7 mW cm −2 ) or a 100-W UV lamp (UVP, LLC; model number B-100AP; light intensity ∼ 10 mW cm −2 ). As a visible light source, we used a fluorescent bulb (light intensity ∼ 1.0 mW cm −2 ). Confocal fluorescence imaging and spectral imaging were performed on an IX81-based Olympus FluoView 1000D laser confocal scanning microscope (Olympus), equipped with a spectral scanning system and two independent laser scanners. To induce SP ring opening, we used light of λ =405 nm. All pictures were collected using a 655–755 nm emission filtre following excitation with a 635-nm laser. To collect emission spectra, we used an excitation wavelength of 405 nm. Preparation of PhotoPAF A single-neck, round-bottom flask with a magnetic stirrer was charged with 4 (51.2 mg; 0.1 mmol; 0.4 mmol of –B(OH) 2 ), 3 (58.7 mg; 0.09 mmol; 0.36 mmol of –Br), 1 (16.05 mg; 0.04 mmol; 0.04 mmol of –Br), Pd(PPh 3 ) 4 (11.6 mg; 0.01 mmol) and potassium carbonate (138.2 mg; 1 mmol). The flask was fitted with a reflux condenser closed with a septum. The reaction mixture was degassed and filled with N 2 , and the procedure was repeated two more times. To the stirred solid mixture under a nitrogen atmosphere, H 2 O (1 ml) was added followed by THF (1 ml), and the reaction mixture was refluxed for 2 days at 75 °C (an additional 1 ml of THF was added after 16 h of reflux). After cooling to room temperature, the reaction mixture was slowly quenched with a concentrated aqueous solution of HCl (1 ml), and the solid residue was filtered. The residue was then washed thoroughly with H 2 O (50 ml), aqueous NaOH solution ( c =1 M; 50 ml), hot H 2 O (70 ml), hot THF (75 ml) and hot CHCl 3 (75 ml). The residue was dried under reduced pressure at 75 °C to yield pure PhotoPAF (60 mg). The procedure described above uses a spiropyran feed ratio, α SP , of 10%. For other PhotoPAFs, relative amounts of 1 and 3 were varied. Actual content of spiropyran in the resulting materials was calculated from elemental analysis data (see Methods). Preparation of PhotoPAN An oven-dried, round-bottom flask with magnetic stirrer was charged with 4 (51.2 mg; 0.1 mmol), 2 (160.1 mg; 0.2 mmol) and Pd(PPh 3 ) 4 (34.7 mg, 0.03 mmol). After adding an aqueous solution of K 2 CO 3 ( c =1 M; 1 ml; 1 mmol), the flask was quickly fitted with a reflux condenser connected to a Schlenk line via a septum. The reaction mixture was degassed, filled with N 2 and the procedure was repeated two more times. THF (4 ml) was added through the septum over the condenser and the reaction mixture was stirred at the reflux temperature (75 °C) under a nitrogen atmosphere for 24 h. After cooling to room temperature, the reaction mixture was slowly quenched with a concentrated aqueous solution of HCl (1 ml), and the solid residue was filtered. The solid residue was then washed thoroughly with H 2 O (75 ml), aqueous NaOH solution ( c =1 M; 75 ml), hot H 2 O (75 ml), hot THF (100 ml) and hot CH 2 Cl 2 (100 ml). The solid product was then suspended in CH 2 Cl 2 (20 ml), sonicated for 1 min and filtered to get PhotoPAN (150 mg), which was then dried under reduced pressure at 75 °C. Calculation of the degree of PhotoPAF substitution To ensure the formation of infinite networks, we use equimolar amounts of the –B(OH) 2 and the –Br groups in the starting materials, the latter originating from both tetrakis(4-bromophenyl)silane 4 and 5′-bromospiropyran 1 —see Supplementary Fig. 37 , where the spiropyran feed ratio, α SP , is defined as the molar ratio of bromospiropyran to the total number of bromoaryl moieties in the starting mixture: We find that in all cases, the content of spiropyran in the final PAFs is lower than that in the initial (‘feed’) mixture. Let us define the content of spiropyran in the final PAFs, χ SP , as the quotient of the number of spiropyran units and the total number of benzene rings originating from Ar–Br: where x < a . To calculate χ SP , we rely on elemental analysis data, and make an assumption that both (silanetetrayltetrakis(benzene-4,1-diyl))tetraboronic acid ( 3 ) and 4 are quantitatively incorporated into the forming PAFs (this assumption is reasonable as each of these substrates has as many as four reactive groups). Let us denote the fraction of residual (unreacted) boronic acid groups in PAFs as y , and the fraction of residual bromine groups as z (see Supplementary Fig. 37 ). Weight percentage of carbon in the final material, % C : where m a, i , atomic mass of element i . Likewise, Solving for x —that is, the molar fraction of SP with respect to 1 in the final PAF—gives: which is related to the actual content of spiropyran in PAFs as and finally, Solid-state NMR studies Solid-state NMR experiments were performed on a 600-MHz Varian VNMRS spectrometer using a triple-channel Varian fastMAS probe. Samples were packed in 1.6 mm rotors for magic angle sample spinning; spinning rate for all experiments was 35,714 Hz, stable to ±10 Hz. For each sample, 1D 1 H and 13 C spectra were collected. All spectra were acquired at room temperature, with sample cooling by application of room temperature air at the probe head. 1 H spectra were acquired using a simple one-pulse sequence, where 32 or 128 scans were collected at a recycle delay of 10 s. 13 C spectra were acquired using the SPIDAP sequence [56] . 13 C-free induction decays were recorded using the 8-π-pulse block repeated 20 or 32 times for an acquisition time 4.5–7 ms per transient, with a recycle delay of 4–8 s (ref. 56 ). 20, 36 and 96 k scans were collected for the 13 C spectra of the small-molecule 2 , PhotoPAF-3.6% and PhotoPAN, respectively. Typical π/2 pulse widths were 0.6 and 1.6 μs for the proton and carbon channels, respectively. Data were processed using ACD/NMR Processor 12.0 (Advanced Chemistry Development, 2007–2010, http:// www.acdlabs.com ). The peak at ∼ 2 p.p.m. seen in the 1 H NMR spectra despite degassing of the samples can be attributed partially to residual solvent, which is corroborated by the following arguments: (i) the peak gradually decreases in spectra collected on consecutive days. For comparison, the peak at ∼ 8 p.p.m. remained constant, (ii) 13 C NMR spectra from initial and final runs looked virtually the same, suggesting that the changes in the 1 H NMR spectra are due to the loss of residual solvent rather than sample decomposition, (iii) PAF prepared without any spiropyran ( y =0 in Fig. 1 ) also shows residual peaks at ∼ 2 p.p.m. ( Supplementary Fig. 30 ), even though its structure only comprises aromatic protons, expected to appear at δ =8 p.p.m., (iv) the peaks attributed to residual solvents seen in the early runs were significantly sharper than other peaks, consistent with the mobile solvent component narrowed by dynamics, which would not be possible for protons attached to the more static carbon skeleton, (v) powder samples often display the presence of solvent molecules [15] , [21] , [22] . Accession codes: The X-ray crystallographic coordinates for structures reported in this article have been deposited at the Cambridge Crystallographic Data Centre (CCDC), under deposition number CCDC 978998. These data can be obtained free of charge from The Cambridge Crystallographic Data Centre via http:// www.ccdc.cam.ac.uk/data_request/cif . How to cite this article: Kundu, P. K. et al. Nanoporous frameworks exhibiting multiple stimuli responsiveness. Nat. Commun. 5:3588 doi: 10.1038/ncomms4588 (2014).